Delivery of endosomes to lysosomes via microautophagy in the visceral endoderm of mouse embryos The differentiation and patterning of murine early embryos are sustained by the visceral endoderm, an epithelial layer of polarised cells that has critical roles in multiple signalling pathways and nutrient uptake. Both nutritional and signalling functions rely upon the endocytosis of various molecules from the cell surface via the endocytic pathway. However, endocytic membrane dynamics in this embryonic tissue remain poorly understood. Here we show that the functions of rab7, a small GTP-binding protein regulating the late endocytic pathway, are essential for embryonic patterning during gastrulation. The endosomes of visceral endoderm cells are delivered via a unique microautophagy-like process to the apical vacuole, a large compartment exhibiting lysosomal characteristics. Loss of rab7 function results in severe inhibition of this endocytic pathway. Our results indicate that the microautophagic process and flow of the endocytic membrane have essential roles in early embryonic development. Mammalian pre-gastrulation embryos are composed of polarised epithelial tissues, an ectoderm and a visceral endoderm (VE; Fig. 1 ) [1] . The VE, which surrounds the epiblast and extraembryonic ectoderm, comprises an absorbing epithelium that supplies nutrients required for embryonic growth [2] , [3] , [4] . VE cells develop numerous microvilli on their apical surfaces and actively internalise various molecules, including transferrin, immunoglobulins (Ig), lipoproteins and albumins [5] , [6] , [7] . 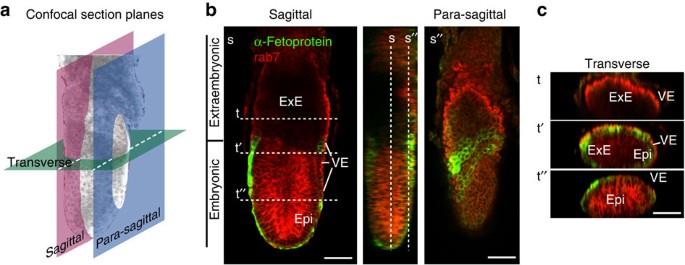Figure 1: Anatomy of mouse E6.2 embryos and interacting tissues. (a) Confocal optical planes of the sagittal, para-sagittal and transverse orientations are shown in pink, blue and green planes, respectively. (b) Wild-type E6.2 embryos were stained for rab7 (red) and α-fetoprotein (green). Serial optical sections of whole mounted embryos were viewed under a laser confocal microscope. Mid-sagittal (S) and para-sagittal (S″) focal planes are shown. (c) Transverse sections (t–t″) were reconstituted from the serial optical sections. The approximate positions of extraembryonic (t), extraembryonic/embryonic junction (t′) and embryonic (t″) sections are indicated in panelb. ExVE cells enveloping the ExE were columnar in shape, whereas the emVE overlying Epi exhibited a squamous morphology. Bars indicate 50 μm. ExE, extraembryonic ectoderm; Epi, epiblast (embryonic ectoderm); VE, visceral endoderm. Figure 1: Anatomy of mouse E6.2 embryos and interacting tissues. ( a ) Confocal optical planes of the sagittal, para-sagittal and transverse orientations are shown in pink, blue and green planes, respectively. ( b ) Wild-type E6.2 embryos were stained for rab7 (red) and α-fetoprotein (green). Serial optical sections of whole mounted embryos were viewed under a laser confocal microscope. Mid-sagittal (S) and para-sagittal (S″) focal planes are shown. ( c ) Transverse sections (t–t″) were reconstituted from the serial optical sections. The approximate positions of extraembryonic (t), extraembryonic/embryonic junction (t′) and embryonic (t″) sections are indicated in panel b . ExVE cells enveloping the ExE were columnar in shape, whereas the emVE overlying Epi exhibited a squamous morphology. Bars indicate 50 μm. ExE, extraembryonic ectoderm; Epi, epiblast (embryonic ectoderm); VE, visceral endoderm. Full size image In addition to its nutritional roles, the VE is essential for embryonic patterning via orchestration of multiple signalling cascades, including transforming growth factor-β (nodal, Wnt, bone morphogenetic proteins (BMPs) and fibroblast growth factors [8] . These secreted signalling molecules bind to cell surface receptors, and ligand-receptor complexes relay the signals to downstream intracellular mediators to trigger further cellular events. In principle, the early stage of endocytosis, that is, the internalisation of signalling receptors from the cell surface to early endosomes, is required for transmitting extracellular stimuli to cytoplasmic mediators [9] , [10] , [11] , [12] , [13] , [14] , [15] . The later stages of endocytosis have roles in signal termination by delivering the signalling molecules to digestive compartments [16] , [17] . Although this scenario is well established in cultured cells, the endocytic dynamics have not been well studied in gastrulating embryos in which precise spatiotemporal regulation of multiple signalling cascades is an absolute requirement. The endocytic pathway comprises several distinctive, but dynamically interacting subcellular compartments: recycling endosomes, early endosomes, late endosomes and lysosomes. Communication between these compartments is mostly mediated by small membrane-bound vesicles that bud from the donor compartment, and then translocate to their destined acceptor compartments, where the vesicular membranes and target membranes fuse to form a continuous membrane, and mixing of luminal contents occurs. In macroautophagy, autophagosome, a double-membrane organelle that engulfs a portion of the cytosol and organelles, fuses with lysosomes to deliver its cargos to digestive compartments. During these delivery processes, membranes of the vesicles or autophagosomes fuse with the distinct membranes of the destination compartments to form continuous membranes. Hereafter, we refer to this mode of membrane interaction as canonical membrane fusion. Cargo delivery may occur via a completely different mechanism known as microautophagy, in which lysosomes take up other organelles and/or cytosol directly by encircling the targets with lysosomal membrane. In yeast cells, peroxisomes are degraded via microautophagy in response to nutrient availability [18] . Mitochondria are also well-known substrates for microautophagic degradation [19] . In mammalian cells, however, the mechanism, and even the phenomenology of microautophagy has not been fully established [20] . In this study, we characterise the endocytic apparatus in the VE of gastrulating mouse embryos. We find that proper endocytic operation towards the terminal compartment requires the function of the small GTP-binding protein rab7. Knockout of rab7 results in severe alterations in the morphology of endocytic compartments and simultaneously causes defects in embryogenesis. Furthermore, endocytic delivery in the VE cells occurred via microautophagy-like membrane dynamics. Endocytic organelles in the VE Cells constituting the developing embryos have different challenges than well-studied mature cells to organise their endocytic membrane system while they maintain the signalling cascades and fulfil the nutritional requirements. We thus analysed the endocytic system in the developing mouse embryos of embryonic day (E) 6.2. The VE cells enveloping the extraembryonic ectoderm (referred to as exVE hereafter) developed extensive microvilli and reticular–vesicular structures, apical canaliculi, beneath the apical plasma membrane ( Fig. 2a ) [21] . Large vacuolar structures (apical vacuoles) were prominent on the apical side of the nuclei ( Fig. 2a , asterisk) and often contained spherical bodies of showing varying brightness under an electron microscope ( Fig. 2a , arrows). By contrast, the VE overlying the epiblast were squamous in shape and the apical vacuoles were smaller ( Fig. 2a , lower panel) [21] . 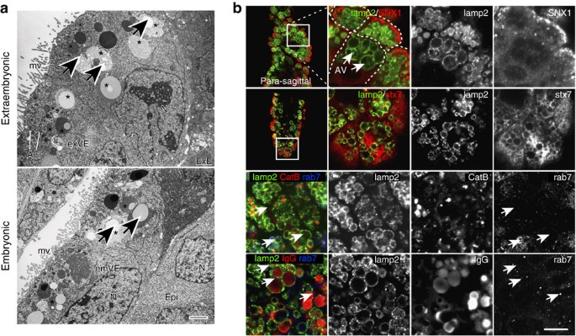Figure 2: Endocytic compartments in the visceral endoderm cells. (a) The morphologies of the cuboidal/columnar cells of the visceral endoderm overlying the extraembryonic ectoderm (exVE) and that of squamous cells covering the epiblast (emVE) are shown. Large apical vacuoles (*) were well developed in the exVE cells. Spherical bodies often appeared inside the apical vacuoles (arrows). Epi, epiblast; mv, microvilli; N, nucleus; VE, visceral endoderm; AC, apical canaliculi; AV, apical vacuoles. Bar: 2 μm. (b) Subcellular localisation of various marker proteins was observed in the VE overlying the extraembryonic ectoderm. Para-sagittal optical sections crossing the VE cell layer (seeFig. 1S″) are shown. The early endosome and late endosome marker proteins, sorting nexin-1 (SNX1) and syntaxin-7 (stx7), respectively, were stained with specific antibodies. The lysosome marker protein, cathepsin B (CatB), was localised in the apical vacuoles whose limiting membranes were positive for lamp2. Immunoglobulin (IgG) of maternal origin was accumulated in the apical vacuoles decorated with lamp2. Single-channel images are also shown. The cellular boundaries indicated by the dotted lines vary reflecting the optical sections of cells at different depths due to the convexity of the embryos. Bar: 10 μm. Figure 2: Endocytic compartments in the visceral endoderm cells. ( a ) The morphologies of the cuboidal/columnar cells of the visceral endoderm overlying the extraembryonic ectoderm (exVE) and that of squamous cells covering the epiblast (emVE) are shown. Large apical vacuoles (*) were well developed in the exVE cells. Spherical bodies often appeared inside the apical vacuoles (arrows). Epi, epiblast; mv, microvilli; N, nucleus; VE, visceral endoderm; AC, apical canaliculi; AV, apical vacuoles. Bar: 2 μm. ( b ) Subcellular localisation of various marker proteins was observed in the VE overlying the extraembryonic ectoderm. Para-sagittal optical sections crossing the VE cell layer (see Fig. 1S″ ) are shown. The early endosome and late endosome marker proteins, sorting nexin-1 (SNX1) and syntaxin-7 (stx7), respectively, were stained with specific antibodies. The lysosome marker protein, cathepsin B (CatB), was localised in the apical vacuoles whose limiting membranes were positive for lamp2. Immunoglobulin (IgG) of maternal origin was accumulated in the apical vacuoles decorated with lamp2. Single-channel images are also shown. The cellular boundaries indicated by the dotted lines vary reflecting the optical sections of cells at different depths due to the convexity of the embryos. Bar: 10 μm. Full size image Previous studies show these organelles constitute the endocytic pathway in VE cells of rodent embryos [22] , [23] . We characterised them by staining with a set of marker molecules known as endosome/lysosome residents. Sorting nexin 1, an early endosomes marker protein [24] , was dense in the apical region and less so in the basolateral regions ( Fig. 2b ). Lamp2, a membrane protein localised mainly to lysosomes [25] , decorated the limiting membranes of the apical vacuoles ( Fig. 2b ) [26] . Syntaxin 7 was localised to the lamp2-positive membranes of the apical vacuoles, but it was also positive in more apical regions, indicating that this late endosomal/lysosomal SNARE [27] , [28] was more broadly distributed than lamp2 ( Fig. 2b ). Cathepsin B, a lysosomal proteinase, was localised in the proximity of lamp2 ( Fig. 2b ). The VE internalises IgG from the maternal circulation through endocytosis [29] , [30] , which is readily detectable by staining with anti-mouse IgG antibodies. The internalised IgG accumulated in compartments limited by lamp2-positive membranes ( Fig. 2b ), indicating that it was transported to the apical vacuoles. The presence of IgG, cathepsin B and lamp2 indicated that the apical vacuoles were the compartments of degradation of internalised materials like the lysosomes in normal cells. The members of rab small GTP-binding proteins are key regulators for vesicular transport at various membrane systems. Rab5, an early endosome marker, exhibited dot-like staining mainly in the apical region of the VE cells ( Supplementary Fig. S1 ). Rab7, a small GTP-protein involved in membrane dynamics during the late stages of the endocytic pathway [31] , [32] , appeared as dots in both the apical and basolateral cytoplasm ( Fig. 2b ). Rab7 signals were often very close to the lamp2-positive membranes and sometimes appeared inside the lamp2-positive compartments ( Fig. 2b , arrows). Membrane dynamics of the endocytic pathway in VE cells Then we examined endocytic activity of VE cells using tracer molecules. The mouse embryos took up fluorescent dextran from the maternal circulation, when the marker dye was intravenously introduced into pregnant mothers ( in utero labelling). Similarly, the embryos dissected from the deciduae can be labelled by the fluorescent dextran under appropriate culture conditions. E6.2 embryos were labelled with rhodamine–dextran (RD) in vitro for 15 min, and then incubated for 15 min in the absence of the marker. During this chase incubation, most internalised RD was transported to the apical vacuoles. The embryos were further labelled with fluorescein–dextran (FD) for 5 min and then chased again in the absence of the fluorescent dye. Immediately after the second labelling, FD appeared in disc- or crescent-shaped structures close to the apical cell surface ( Fig. 3a , 0 min, and Supplementary Movie 1 ). The FD-containing compartments and RD-labelled apical vacuoles were often attached to each other, but the red and green signals were well separated. Within the next 5–15 min, the disc-shaped FD compartments became spherical and were frequently surrounded by the RD signal ( Fig. 3a and Supplementary Movies 2,3 ). As seen in the optical sections, FD signals were facing a non-fluorescent region (presumably the cytosolic space) in at least one region ( Supplementary Movies 2,3 ), indicating that the RD-accumulating compartments had not completely engulfed the FD-containing compartments. In addition to the dextran-accumulating compartments, numerous non-fluorescent spherical bodies were observed in the apical vacuoles, producing an image resembling dark cheese eyes in red cheese ( Fig. 3a , 0 min, arrows, and Supplementary Movies 1–3 ). These non-fluorescent bodies were presumably endosomes internalised during the first chase period. Further, mixing of the red (RD) and green (FD) signals occurred during 15–0 min after the second labelling, and most apical vacuoles became yellow ( Fig. 3a , 15 and 30 min). 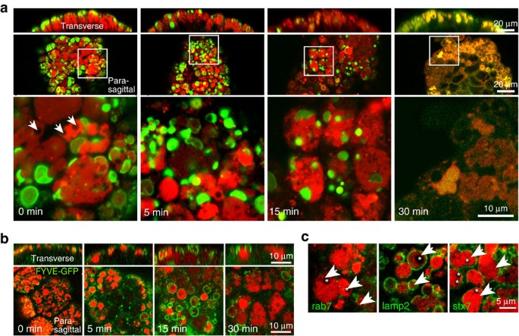Figure 3: Endocytosis of fluorescent dextran in the visceral endoderm. (a) Endocytosis of fluorescent dextran in VE. E6.2 mouse embryos were cultured and labelled with rhodamine dextran (RD) for 15 min, chased for 15 min, pulse labelled with fluorescein dextran (FD) for 5 min, and then chased for the indicated durations. The stained embryos were fixed and serial optical sections were acquired using a laser-scanning confocal microscope. (b) Transient association of PtdIns(3)P with the endosomes in VE. E6.2 mouse embryos from FYVE–GFP transgenic mice were labelled with RD (red) for 15 min and then chased for the indicated durations. The signals of the FYVE–GFP fusion protein, which specifically labelled PtdIns(3)P, are shown in green. (c) Membrane proteins on the endosomes. E6.2 embryos were cultured in DMEM+rat serum and then preloaded with RD for 15 min, chased for 15 min and fixed. The labelled embryos were immunostained with anti-rab7, anti-lamp2 or anti-syntaxin7 (stx7) antibody. The rab7 signals often appeared inside the lamp2-positive compartments (arrows). The cheese-eye like structures (*) were negative for lamp2 and syntaxin-7. Figure 3: Endocytosis of fluorescent dextran in the visceral endoderm. ( a ) Endocytosis of fluorescent dextran in VE. E6.2 mouse embryos were cultured and labelled with rhodamine dextran (RD) for 15 min, chased for 15 min, pulse labelled with fluorescein dextran (FD) for 5 min, and then chased for the indicated durations. The stained embryos were fixed and serial optical sections were acquired using a laser-scanning confocal microscope. ( b ) Transient association of PtdIns(3)P with the endosomes in VE. E6.2 mouse embryos from FYVE–GFP transgenic mice were labelled with RD (red) for 15 min and then chased for the indicated durations. The signals of the FYVE–GFP fusion protein, which specifically labelled PtdIns(3)P, are shown in green. ( c ) Membrane proteins on the endosomes. E6.2 embryos were cultured in DMEM+rat serum and then preloaded with RD for 15 min, chased for 15 min and fixed. The labelled embryos were immunostained with anti-rab7, anti-lamp2 or anti-syntaxin7 (stx7) antibody. The rab7 signals often appeared inside the lamp2-positive compartments (arrows). The cheese-eye like structures (*) were negative for lamp2 and syntaxin-7. Full size image Phosphatidylinositol 3-phosphate (PtdIns(3)P) signalling has a regulatory role in the assembly of late endosomes and lysosomes, as well as in autophagic membrane processes [33] , [34] . The FYVE domain is a zinc-finger motif with high affinity for PtdIns(3)P, and the green fluorescent protein (GFP)–FYVE fusion protein has been widely used for probing subcellular localisation of PtdIns(3)P in living cells [35] . We created a transgenic mouse strain in which the GFP–FYVE fusion protein was expressed under the control of the ubiquitously active, cytomegalovirus immediate early enhancer-chicken β-actin hybrid promoter. Mouse embryonic fibroblasts (MEFs) prepared from the transgenic mice exhibited bright GFP-signals dispersed in the cytoplasm. When the MEFs were fed with an endocytic marker Alexa Fluor 555-conjugated bovine serum albumin, the GFP signals were well colocalised with the endocytic marker immediately after labelling. After a 4-h chase, the GFP- and Alexa-bovine serum albumin signals became separated ( Supplementary Fig. S2 ), indicating that the GFP–FYVE fusion protein was successfully identified as the PtdIns(3)P positive, early endocytic compartments. Next, we labelled the embryos of the transgenic mouse with RD for 15 min in the embryo culture medium. In the early phase of endocytosis, the GFP signals gradually accumulated at the rim of the RD compartments, which often appeared as disc- or crescent-shaped structures ( Fig. 3b , 0 to 5-min chase), and then surrounded the round medium-sized organelles ( Fig. 3b , 15-min chase). However, only a few GFP signals became associated with the large RD compartments after a 30-min chase. This observation suggested that PtdIns(3)P was transiently associated with the endosomes. Consistent with this observation, the genetic loss of a PtdIns(3)P metabolising enzyme PIPKIII results in severe defects in the apical vacuole morphogenesis (our unpublished observation). As described above, we frequently found rab7 inside lamp2 rings ( Fig. 2b ). In the RD-labelling experiments, rab7 often appeared at the interfaces between the RD-positive areas and the dark 'cheese eyes', confirming that rab7-positive membranes were internalised by the apical vacuoles ( Fig. 3c ). Stx7 and lamp2 were localised to the limiting membrane of the apical vacuoles, but they were not seen at the rims of the internalised endosomes, suggesting that the apical vacuolar membrane surrounding the endosomes had a distinct membrane composition ( Fig. 3c ). Endosomes are engulfed by vacuoles via a microautophagy During visualisation of endocytic markers in the embryos, we noted that the microscopic images appeared as though the endosomes were engulfed by the apical vacuoles ( Fig. 3a ). Fusion of the limiting membranes of endosomes and apical vacuoles to form a continuous membrane (canonical fusion) would lead to mixing of the contents of the endosomes with those of the apical vacuoles. However, the endocytic marker images suggested that this was unlikely. Three-dimensional analysis of the confocal images showed that the dextran-loaded endosomes inside the apical vacuoles existed as spherical bodies ( Supplementary Movie 3 ). We examined the RD/FD compartments in live embryos cultured in vitro . The RD-labelled spherical body (as well as dark, non-labelled bodies) moved around in the FD-pre-labelled apical vacuoles for several minutes before mixing, and then it disappeared within 30 s ( Supplementary Movie 4 ). A z axis scan showed that the RD-signal merged with the FD-signal, rather than going out of focus ( Fig. 4a,b ). 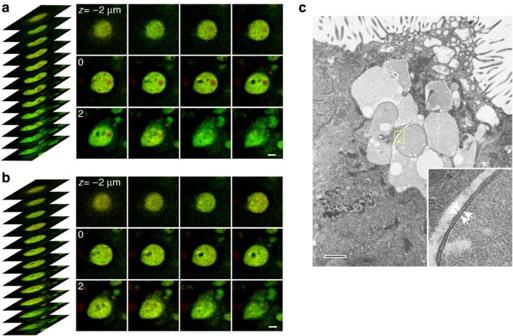Figure 4: Characterisation of the endocytic pathway in the visceral endoderm cells. (a,b) RD-loaded spherical body disintegrates inside the apical vacuole. E6.2 embryos were cultured in DMEM+rat serum and preloaded with FD, then pulse labelled with RD. Optical sections of the spherical body shown inSupplementary Movie 4were arranged before (a) and after (b) the disappearance of the RD signal. Panelsaandbcorrespond to the time points 07:30 and 08:00 h in theSupplementary Movie 4. Bars indicate 2 μm. (c) Membranes surrounding the spherical bodies in apical vacuoles. E6.2 mouse embryos were fixedin uteroand then processed for electron microscopy. Double membranes (arrows) encircled the spherical bodies. Apical vacuoles were observed in VE cells overlying ExE were observed. Bar indicates 1 μm. Figure 4: Characterisation of the endocytic pathway in the visceral endoderm cells. ( a , b ) RD-loaded spherical body disintegrates inside the apical vacuole. E6.2 embryos were cultured in DMEM+rat serum and preloaded with FD, then pulse labelled with RD. Optical sections of the spherical body shown in Supplementary Movie 4 were arranged before ( a ) and after ( b ) the disappearance of the RD signal. Panels a and b correspond to the time points 07:30 and 08:00 h in the Supplementary Movie 4 . Bars indicate 2 μm. ( c ) Membranes surrounding the spherical bodies in apical vacuoles. E6.2 mouse embryos were fixed in utero and then processed for electron microscopy. Double membranes (arrows) encircled the spherical bodies. Apical vacuoles were observed in VE cells overlying ExE were observed. Bar indicates 1 μm. Full size image Electron microscopic images also supported the scenario that the apical vacuoles engulfed the endosomes. Double membranes encircled the spherical bodies inside the apical vacuoles, presumably one being the limiting membrane of the apical vacuole and the other that of the endosome itself ( Fig. 4c and Supplementary Fig. S3 ). Three-dimensional reconstructions generated from confocal sections showed that the endosomes were completely engulfed by the apical vacuoles and lost their connection to the cytosol ( Supplementary Movie 5 ). In addition, serial sections of electron microscopy also confirmed that the limiting membrane was pinched off from the limiting membrane of the surrounding apical vacuoles ( Fig. 5 and Supplementary Movies 6, 7 ). 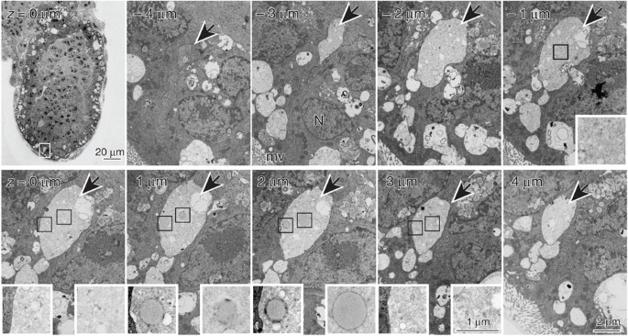Figure 5: Serial sections of apical vacuoles in the visceral endoderm. E6.0 mouse (ICR) embryos were fixedin uteroand processed for electron microscopy. Serial sections were prepared at 1-μm intervals and viewed under an electron microscope. The large apical vacuole is indicated by arrows and two spherical bodies are shown in black squares. Higher magnification images of the spherical bodies are also shown. Figure 5: Serial sections of apical vacuoles in the visceral endoderm. E6.0 mouse (ICR) embryos were fixed in utero and processed for electron microscopy. Serial sections were prepared at 1-μm intervals and viewed under an electron microscope. The large apical vacuole is indicated by arrows and two spherical bodies are shown in black squares. Higher magnification images of the spherical bodies are also shown. Full size image Lipase-dependent mixing of endosome–vacuole contents If the endosomes were delivered to the apical vacuoles via an orthodox process involving the canonical membrane fusion, the endosomal and vacuolar contents would eventually mix even in the absence of lipase activity. However, delivery of endosomes occurred via a mechanism involving engulfment of endosomes by the apical vacuoles: therefore, mixing of the materials inside the endosomes with those in apical vacuoles required membrane disintegration. In yeast vacuoles, disintegration of autophagic bodies requires the function of Aut5/Cvt17, a protein with a lipase motif [36] , [37] . We examined whether lipase activity was required for the contents mixing. The embryos were sequentially labelled with RD and FD, and chased in the presence of tetrahydrolipstatin (orlistat), an irreversible inhibitor of lysosomal acid lipases [38] . The RD and FD signals mixed after 15-min incubation in the absence of the inhibitor ( Fig. 3a ). The lipase inhibitor prevented the mixing of the contents, leaving the RD and FD signals well separated even after 30 min of incubation ( Fig. 6 ). The RD was detected in the apical vacuoles, whereas FD was detected as smaller spherical bodies inside the apical vacuoles, producing green 'cheese-eyes' in red 'cheese' images ( Fig. 6 , arrows). Non-labelled 'cheese-eyes' ( Fig. 6d,e , asterisk) frequently appeared in the apical vacuoles treated with the lipase inhibitor and they most likely reflected the endosomes formed after the FD had been washed out. This finding indicated that orlistat did not affect the internalisation or endosome formation, but prevented the mixing of the contents of endosomes and apical vacuoles. Further, orlistat did not interfere with the mixing of the first and second endocytic markers in the NIH3T3 cells in which the major endocytic pathway proceeds via the canonical fusion ( Supplementary Fig. S4 ). 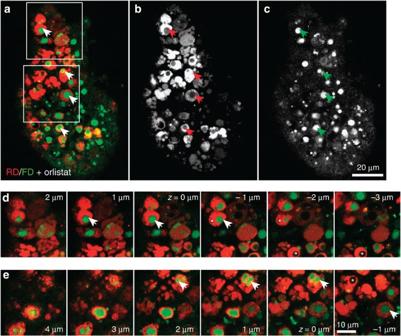Figure 6: Effect of lipase inhibition on the endosome-apical vacuole interaction. (a) E6.2 embryos were pre-labelled with RD, and then labelled with FD and chased for 30 min in the presence of the lipase inhibitor tetrahydrolipstatin (orlistat), and observed under a confocal microscope. The RD signal (a,b) was well separated from the FD signal (a,c) that appeared inside the red-stained compartments. Panelsdandeshow different focal planes (z=1 μm) of the squared areas in panela. Figure 6: Effect of lipase inhibition on the endosome-apical vacuole interaction. ( a ) E6.2 embryos were pre-labelled with RD, and then labelled with FD and chased for 30 min in the presence of the lipase inhibitor tetrahydrolipstatin (orlistat), and observed under a confocal microscope. The RD signal ( a , b ) was well separated from the FD signal ( a , c ) that appeared inside the red-stained compartments. Panels d and e show different focal planes ( z =1 μm) of the squared areas in panel a . Full size image Delivery of endosomes to vacuoles requires rab7 function The rab7 protein functions in the late stages of the endocytic pathway as an essential regulator of vesicular trafficking and macroautophagy [31] , [32] . Indeed, the rab7 protein is abundantly expressed in the pre-gastrulation embryos and is localised to the apical vacuoles of the VE ( Figs 1 , 2 , 3 ). To investigate the roles of rab7 in developing embryos, we generated mutant mice harbouring a rab7 -null allele ( Supplementary Fig. S5 ). In the VE of E6.2 rab7 -deficient embryos, large apical vacuoles were absent. Instead, accumulation of smaller, fragmented vesicles was observed ( Fig. 7a ). The rab7 -deficient VE cells were defective in the endocytic pathway. Some of the fragmented vesicles were positive for lamp2, but the majority of internalised IgG derived from the maternal circulation did not clearly overlapped with lamp2 ( Fig. 7b,c ). In addition, the mutant cells effectively internalised the dextrans in the culture medium; however, RD and FD remained spatially separated in the cytoplasm ( Fig. 7d ). These observations indicated that rab7 function is required for the merging of the endosomes. 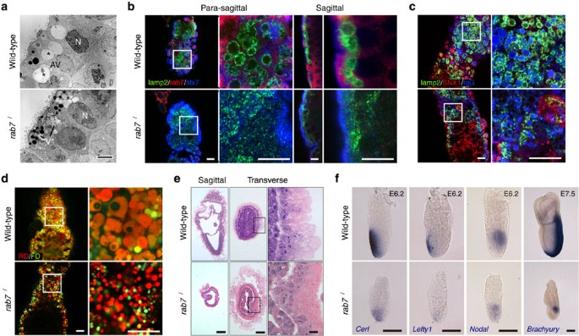Figure 7: Rab7 function is required for the endocytic pathway and embryogenesis. (a) Electron micrographs of the VE of E6.5 wild-type andrab7−/−embryos. The wild-type cells developed prominent apical vacuoles (AV, indicated by *), whereas the mutant cells accumulated heterogeneously stained fragmented organelles. Bar indicates 5 μm. (b) Localisation of lamp2 (green), rab7 (red) and syntaxin7 (stx7, blue) in VE cells of E6.2 embryos. The red signal for rab7 was absent in therab7−/−embryo. Bar indicates 15 μm. (c) Localisation of lamp2 (green), sorting nexin 1 (SNX1, red) and endogenous immunoglobulin taken up from maternal circulation (IgG, blue) in VE cells of E6.2 embryos. The IgG signals were detected in the VE cells, but most of them did not overlap with the lamp2 signals in therab7−/−embryo. Bar indicates 15 μm. (d) Endocytosis of fluorescent dextran in the VE ofrab7mutant embryos. The embryos were labelled with RD (red) for 15 min, chased for 15 min, pulse labelled with FD (green) for 5 min, and then chased for 30 min. Bar indicates 15 μm. (e) Morphology of rab7-deficient embryos. Mouse embryos were dissected at E7.5, embedded in Technovit 7100 resin, and sagittal and transverse section were stained with haematoxylin and eosin. Bars indicate 100 μm in sagittal, 50 μm in transverse, and 10 μm in enlarged images. (f) Expression patterns of various marker genes by whole-mountin situhybridization. AVE markersCerlandLefty-1,Nodal, and a mesoderm markerBrachyurywere analysed by whole-mountin situhybridisation. Bar indicates 100 μm. Figure 7: Rab7 function is required for the endocytic pathway and embryogenesis. ( a ) Electron micrographs of the VE of E6.5 wild-type and rab7 −/− embryos. The wild-type cells developed prominent apical vacuoles (AV, indicated by *), whereas the mutant cells accumulated heterogeneously stained fragmented organelles. Bar indicates 5 μm. ( b ) Localisation of lamp2 (green), rab7 (red) and syntaxin7 (stx7, blue) in VE cells of E6.2 embryos. The red signal for rab7 was absent in the rab7 −/− embryo. Bar indicates 15 μm. ( c ) Localisation of lamp2 (green), sorting nexin 1 (SNX1, red) and endogenous immunoglobulin taken up from maternal circulation (IgG, blue) in VE cells of E6.2 embryos. The IgG signals were detected in the VE cells, but most of them did not overlap with the lamp2 signals in the rab7 −/− embryo. Bar indicates 15 μm. ( d ) Endocytosis of fluorescent dextran in the VE of rab7 mutant embryos. The embryos were labelled with RD (red) for 15 min, chased for 15 min, pulse labelled with FD (green) for 5 min, and then chased for 30 min. Bar indicates 15 μm. ( e ) Morphology of rab7-deficient embryos. Mouse embryos were dissected at E7.5, embedded in Technovit 7100 resin, and sagittal and transverse section were stained with haematoxylin and eosin. Bars indicate 100 μm in sagittal, 50 μm in transverse, and 10 μm in enlarged images. ( f ) Expression patterns of various marker genes by whole-mount in situ hybridization. AVE markers Cerl and Lefty-1 , Nodal , and a mesoderm marker Brachyury were analysed by whole-mount in situ hybridisation. Bar indicates 100 μm. Full size image Genetic loss of the rab7 function resulted in the embryonic lethality around E7–8; the mesoderm was not properly organised and the embryos remained as egg cylinders ( Fig. 7e ). Before the gastrulation, the rodent embryos establish the anterior–posterior axis, which can be molecularly visualised by the expression of specific genes like Cerl and Lefty-1 ( Fig. 7f ). At E6.2, mouse embryos establish the anterior VE (AVE), a specific repertoire of the VE [39] . The AVE expresses and secretes the Cerl and Lefty-1, which suppress Nodal signalling in the epiblast. Nodal signalling is required for the differentiation of the mesoderm from a subset of embryonic ectoderm, and therefore, the mesoderm Brachyury expression in the nascent mesoderm. In the mutant, the expression of Cerl , an AVE marker gene was much weaker than that of wild-type embryos ( Fig. 7f ). In addition, the mutant embryos expressed much reduced amounts of another AVE marker, Lefty-1 . Their products, Cerl and Lefty-1, are secreted from the AVE and suppress Nodal expression in the epiblast close to the AVE, thereby restricting the Nodal -expressing domain to the posterior side [40] . In the rab7 mutant, this posterior restriction of Nodal expression was less obvious ( Fig. 7f ). The mutant embryos initiated the expression of a nascent mesoderm marker Brachyury in the proximal, posterior region of the epiblast, thereby enabling the establishment of the anterior–posterior axis at the beginning of gastrulation ( Fig. 7f ). This implies that the defects in signalling patterns may be rather quantitative. Nevertheless, the mutant embryos could not elongate the primitive streak along the midline and failed to complete gastrulation ( Fig. 7e,f ). Thus, rab7 -dependent endocytosis is essential in this early developmental stage. The VE cells actively internalise endocytic markers. The internalised materials are delivered to the apical vacuoles, which are the most prominent organelles with lysosomal characteristics in VE cells. Not only their appearance, but also their membrane dynamics, involving the microautophagic process is unique ( Fig. 8 ). Bulk uptake of external and/or cell surface materials via endocytosis simultaneously delivers the components of the plasma membranes to late endosomes and lysosomes, leading to transfer of membrane components from the cell surface to intracellular compartments. Besides endocytic delivery, biogenetic flow from the Golgi apparatus continuously supplies membranes to the apical vacuoles, which should also be balanced by mechanisms such as membrane traffic from the lysosome to the Golgi apparatus. Microautophagy of endosomes delivers the membranes of both plasma membrane/endosome and lysosome/vacuole origins into the lumen of the apical vacuoles where digestive enzymes including lipases are abundant [41] . Consequently, this microautophagic process does not increase, but rather decreases the surface area of the apical vacuoles. The unique membrane dynamics in VE cells may participate in maintaining their organelle size and integrity despite the extensive endocytosis to sustain nutritional requirements. 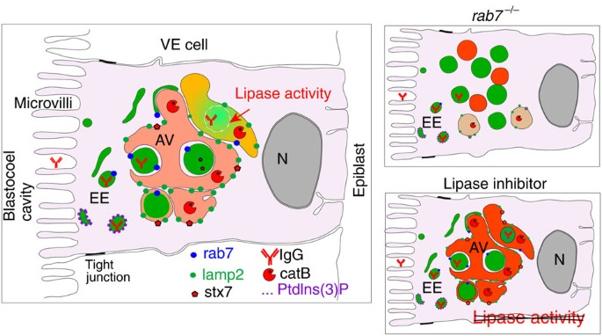Figure 8: Membrane dynamics in visceral endoderm cells. Endocytosed molecules are transported from the cell surface to the apical vacuolesviaearly endosomes and spherical bodies in VE cells. Apical vacuoles engulf endosomes by inwardly invaginating their limiting membranes. The surrounding membranes, which were originally the limiting membranes of the apical vacuoles, are then digested by lipases inside the apical vacuoles. Finally, the endosomal membranes (internalised inside the apical vacuoles) disintegrate, and the endosomal contents appear in the lumen of the apical vacuoles. This process is topologically similar to microautophagy. In therab7mutant embryo, endosomes remained as distinct smaller compartments, indicating that the rab7 function is required for the merging of endosomes. AV, apical vacuole; catB, lysosomal proteinase cathepsin B; EE, early endosome; N, nucleus; PtdIns(3)P, phosphatidylinositol 3-phosphate; stx7, syntaxin-7. Figure 8: Membrane dynamics in visceral endoderm cells. Endocytosed molecules are transported from the cell surface to the apical vacuoles via early endosomes and spherical bodies in VE cells. Apical vacuoles engulf endosomes by inwardly invaginating their limiting membranes. The surrounding membranes, which were originally the limiting membranes of the apical vacuoles, are then digested by lipases inside the apical vacuoles. Finally, the endosomal membranes (internalised inside the apical vacuoles) disintegrate, and the endosomal contents appear in the lumen of the apical vacuoles. This process is topologically similar to microautophagy. In the rab7 mutant embryo, endosomes remained as distinct smaller compartments, indicating that the rab7 function is required for the merging of endosomes. AV, apical vacuole; catB, lysosomal proteinase cathepsin B; EE, early endosome; N, nucleus; PtdIns(3)P, phosphatidylinositol 3-phosphate; stx7, syntaxin-7. Full size image Microautophagy is thought to be a 'non-selective' process by which lytic compartments engulf a portion of the cytosol [42] . In this regard, the structures observed in the VE appeared to be selective for endosomes with minimum amounts of cytosol, judging from the electron micrographs and fluorescence images. The endosome-apical vacuole interaction resembled pexophagy in yeast cells, by which peroxisomes are internalised by digestive vacuoles in response to the nutritional conditions [18] . Endocytic uptake of the extraembryonic materials by VE cells provides nutritional supplies and is required for the functions of multiple signalling cascades. The early stages of endocytic pathway constitute the subcellular platforms where the extracellular stimuli are transmitted to the cytosolic effectors. This endosomal function as a signalling centre has been shown for various ligand-receptor systems, including Wnt, transforming growth factor-β, BMP and fibroblast growth factor, which have central roles in embryonic patterning. Mutations affecting the early stages of the endocytic pathway caused various developmental abnormalities [43] , [44] . In contrast to these promoting roles of the early endosomes in the signal transduction, the late stages of the endocytic pathway can terminate signalling events by separating the activated receptors from cytosolic transducers. This function should be quite important, particularly in the peri-gastrulation embryos, where cell–cell interactions via signalling molecules occur in a highly ordered sequence even in a short period. Thus, the duration of events is highly regulated by several means to fulfil the spatiotemporal requirements of the signalling. Rab7-deficency caused dramatic alteration in the endocytic compartments. In yeast, loss of Ypt7p (the rab7 counterpart in yeast) results in fragmentation of vacuolar compartments [45] , [46] . A similar phenotype was seen in the mouse embryos upon the genetic inactivation, confirming that the basic molecular logic operating in the endocytic pathways are well conserved in the evolutionarily distant species, such as yeast and mouse. Mouse mutants defective in the vacuole assembly exhibited the embryonic lethality around gastrulation. We speculate that the normal endocytic pathway is certainly involved in the regulation of signalling cascades. This scheme is consistent with evidence from several genetic studies. Disassembly of apical vacuoles occurs in cubilin-deficient embryos [47] . Cubilin and its co-factor amnionless act as an endocytic receptor for multiple-ligands [48] . As suggested by the name, the embryos lacking amnionless exhibit defective gastrulation, with severe disorganisation of the embryonic ectoderm and embryonic mesoderm. The cubilin mutant exhibits a developmental defect similar to that of the amnionless mutant [47] , [49] . Loss of function of p18, a lipid raft adaptor essential for the MEK–ERK pathway and mammalian target of rapamycin complex 1 signalling, results in a similar phenotype to that of amnionless [26] . Further, we showed most recently that the spatio-temporal patterns of BMP/Smad1 signalling are controlled by mVam2-dependent membrane trafficking to the apical vacuole [50] . These observations imply that the proper assembly of the apical vacuoles is essential for regulating morphogenetic signalling cascades and normal progress of gastrulation. Animals All animal experiments were approved by the institutional committee (ISIR, Osaka University), and were carried out in accordance with the rules and regulations of the institutions and the government. C57Bl/6 and ICR mice were purchased from SLC, Japan. The animals were supplied with food and water ad libitum . Rab7 mutant mice were generated by embryonic stem cell-mediated gene targeting (R1, kindly provided by A. Nagy) [51] . A targeting vector was created using the recombinogenic strategy [52] . A bacterial artificial chromosome clone (bMQ423o22) was provided from Wellcome Trust Sanger Institute and introduced into an Escherichia coli strain DY380 carrying an inducible homologous recombination system [52] . A lox P-Zeo- lox P fragment was amplified by PCR using a pair of primers (Rab7-LZL forward: 5′-ggttgtccctaaacagagttgcactgtgaagcattgttcatcctccagtctcatgtttgataattctttaCACATCTCAACCATCATCGATCATAA-3′ and Rab7-LZL reverse: 5′-atatatatattctccactttctaaaattctccatgaggacagttttgttttctatttgcctggtgccaagACACATCTCAACCCTGAAGCTATCATAA-3′; lowercase letters correspond to sequences in intron 1–2 of the rab7 locus, and uppercase letters correspond to pMODloxZeo-Δamp3, the lox P-Zeo- lox P cassette vector [53] ), and introduced into bMQ423o22/DY380. Next, a linear pBSDT-AII fragment [53] flanked by short rab7 segments was amplified by primers Rab7DTA1: 5′-tactcccaaccccaccgtcccagagtctgtgttgactcagcaaggtttcagtctcactgaagatcTCCGGCCGGCCCGGGCGATCCCCCG-3′ and Rab7DTA2: 5′-caggccttccagacaattgctcggaatgcccttaaacaggtgggtctcagggccctcaagctgcaTCCTAGAGCGGCCGCCACCGCGGTC-3′ (lowercase and uppercase letters correspond to rab7 and pBSDT-AII sequences, respectively), and introduced into DY380 carrying the modified bacterial artificial chromosome to retrieve an approximately 12-kb fragment in the multicopy plasmid pBSDT-AII. The resultant plasmid was further modified with a lox P- Frt - npt - lox P- Frt cassette using a mini-transposon-mediated strategy to yield a targeting vector in which the lox P- Frt - npt - lox P- Frt was placed into intron 3–4, and the third lox P into the intron 1–2 ( Supplementary Fig. S5 ). Cre-mediated recombination between the remotest lox P sequences [54] , [55] produced an allele missing the exons 2 and 3, which encode the amino acid residues 1–133 of 207. EEA1–FYVE–GFP transgenic mice were generated by pronuclear injection of a DNA fragment of the cytomegalovirus enhancer/β-actin promoter fused to the FYVE domain of the EEA1 protein and GFP (RBRC01161 or RBRC01162 at RIKEN BioResource Centre). MEFs were obtained from E12.5 embryos by standard methods [56] and cultured in DMEM containing 10% fetal bovine serum. Immunofluorescence labelling of the embryos Embryos were obtained from pregnant females killed either by cervical dislocation (for embryo culture) or by fixative perfusion (4% paraformaldehyde (PFA) in PBS) under pentobarbital anaesthesia. For immunohistochemistry, the fixed embryos were incubated with primary and the secondary antibodies in a blocking solution containing 0.05% Tween-20, 0.5% TSA blocking reagent (PerkinElmer) and 1% normal donkey serum in PBS. Affinity-purified rabbit anti-sorting nexin 11, anti-rab7 and anti-syntaxin 7 antibodies [24] , [28] were used at 2.4, 15 and 4.1 μg ml −1 , respectively, in the blocking solution. Anti-rab7 monoclonal antibodies (chicken) [50] were used at 6.9 μg ml −1 . Anti-lamp2 monoclonal antibodies (rat) were obtained from Developmental Study Hybridoma Bank, and used at 4.4 μg ml −1 . Anti-cathepsin B (rabbit) and anti-rab5 (rabbit) were from Upstate and Stressgen, used at 5.0 and 2.5 μg ml −1 , respectively. Fluorescein-, Cy3- and Cy5-conjugated secondary antibodies were obtained from Jackson ImmunoResearch, reconstituted in 50% glycerol according to the manufacturer's recommendation, and used at 1:100, 1:500 and 1:250 dilution, respectively, in the blocking solution. Whole-mount in situ hybridisation was performed by a standard method using digoxigenin-labelled probes [57] . Embryos were staged according to the dissection time (noon of the vaginal plug as E0.5) and morphology. Embryo culture and endocytic labelling Deciduae were dissected out from E6.2 pregnant females killed by cervical dislocation, and placed in DMEM containing 10% fetal bovine serum and 25 m M HEPES (pH 7.5). Embryos were dissected in the same medium under a stereomicroscope, and cultured in a 1:1 mixture of DMEM and rat serum under 5% CO 2 and 95% air at 37 °C [58] . The embryos were incubated with fluorescent dextran (2 mg ml −1 ) in the culture medium for the indicated durations, and then washed with the culture medium twice. After the final labelling and chase, the embryos were transferred to ice-cold 4% PFA/PBS and fixed overnight at 4 °C, and then processed for immunostaining or observed under a laser-scanning confocal microscope (Zeiss LSM510). For orlistat treatment, the RD-labelled embryos were pulse labelled with FD, chased for 30 min in a medium containing orlistat (5 μg ml −1 ) and processed for microscopy. For lamp2 detection using rat monoclonal antibodies, the embryos were labelled in utero by administering 200 μl of 1 mg ml −1 RD in mouse-tonic saline intravenously via the lateral tail-vein of a pregnant mother, and the embryos were dissected and then processed for immunofluorescence labelling as described above. For live imaging ( Fig. 3b,c and Supplementary Movie 4 ), the culture was placed on a Leica ASMDW microscope equipped with a humidified chamber (5% CO 2 , 95% air, 37 °C) and the images were acquired and processed with Leica ASMDW and DeBlur software. Microscopy Embryos were mounted in 0.1% gellan gum (Sigma-Aldrich) in PBS containing 40% glycerol and 0.2% Tween 20 in a glass-bottom 35 mm dish, and then viewed under a confocal laser-scanning microscope (Zeiss LSM510) or a wide-field fluorescence microscope (Leica ASMDW). The images were processed for presentation with Adobe Photoshop CS4, Illustrator CS4 and GoLive software on Macintosh computers. For electron microscopy, embryos were fixed with 2% glutaraldehyde and 2% PFA in 0.1 M potassium phosphate (pH 7.2), and then processed according to standard procedures [59] , [60] . Electron microscopy was performed at the Hanaichi Ultra-Structure Research Institute (Okazaki, Japan). Reagents Tetramethylrhodamine- and fluorescein-conjugated dextrans (MW 70,000, aldehyde fixable) were purchased from Invitrogen. Tetrahydrolipstatin (Orlistat) was purchased from LKT Laboratories. How to cite this article: Kawamura, N. et al . Delivery of endosomes to lysosomes via microautophagy in the visceral endoderm of mouse embryos. Nat. Commun. 3:1071 doi: 10.1038/ncomms2069 (2012).